Spatial extent of a Landauer residual-resistivity dipole in graphene quantified by scanning tunnelling potentiometry Electronic transport on a macroscopic scale is described by spatially averaged electric fields and scattering processes summarized in a reduced electron mobility. That this does not capture electronic transport on the atomic scale was realized by Landauer long ago. Local and non-local scattering processes need to be considered separately, the former leading to a voltage drop localized at a defect, the so-called Landauer residual-resistivity dipole. Lacking precise experimental data on the atomic scale, the spatial extent of the voltage drop remained an open question. Here, we provide an experimental study showing that the voltage drop at a monolayer–bilayer boundary in graphene clearly extends spatially up to a few nanometres into the bilayer and hence is not located strictly at the structural defect. Moreover, different scattering mechanisms can be disentangled. The matching of wave functions at either side of the junction is identified as the dominant process, a situation similar to that encountered when a molecule bridges two contacts. The description of electron transport requires paradigms bridging all length scales from atomic to sample dimensions. As a result, most conductivity measurements include a variety of very different scattering mechanisms that could typically be disentangled only by theory. Moreover, most of our electronic devices today are characterized by a global conductivity or mobility of carriers which are often described with semiclassical concepts of transport, for example, the Boltzmann equation. That electron propagation through a sample has to be described by quantum mechanics becomes apparent only in cleverly designed experiments, for example, as universal conduction fluctuations, conductance quantization and the quantum Hall effect [1] . These experiments and the corresponding theoretical description constitute the wealth of collected knowledge on the topic mesoscopic transport. In contrast, non-equilibrium phenomena of electronic transport on the atomic scale are less well explored experimentally. Such measurements have been carried out at two-dimensional conductors [2] , [3] , graphene being a recent prominent system [4] , [5] , [6] , [7] , [8] . The experiments demonstrated the influence of non-local scattering processes (for example, electron–phonon or electron–electron scattering) in defect-free sample regions as well as electron scattering at localized defects like steps, interfaces and grain boundaries. Scattering at these defects was up to now only observed as localized discontinuities in the voltage drop, that is, experiments did not resolve the shape of the potential across a localized scatterer. The answer to the simple question, ‘Where does the voltage drop occur?’ is of specific interest as it gives access to the inherently non-equilibrium quantum mechanical processes. In the following, we show that the voltage drop at a monolayer–bilayer(ML–BL) interface in graphene extends several nanometres into the bilayer. This is in contrast to the situation at substrate steps covered with ML graphene and in contrast to previous reports. We conclude that this effect is caused by the electronic coupling within the transition region to the electron reservoir of the ML or BL side. In this sense, the transition region bridges two electron reservoirs similar to a molecule in transport across molecular break junctions [9] , [10] . We further demonstrate that different scattering mechanisms can be distinguished revealing the rather small influence of the detachment of the graphene layer from the substrate step. The monolayer–bilayer interface in epitaxial graphene Using scanning tunnelling potentiometry (STP) [11] at 6 K (see Fig. 1a ), we demonstrate that the spatial characteristics of the voltage drop can be resolved with sub-nanometre resolution. At the atomic scale, a current flowing across a structural defect leads to the accumulation of electrons on one and depletion on the other side. This Landauer residual-resistivity dipole [12] is caused by the reduced transmission probability of the electrons past a defect. Consequently, the electrochemical potential (ECP) changes locally leading to the observed voltage drop [1] , [13] , [14] , [15] , [16] . In the case of one-dimensional defects in a two-dimensional conductor, an interesting parallel can be drawn to electron transport through single molecules [9] , which has been theoretically studied in great detail in the past. According to Xue and Ratner [10] , the change in the ECP occurs over the length of the molecule since different molecular orbitals couple differently to the electron reservoirs at the end of the molecule. The ML–BL junction in graphene [17] on silicon carbide (SiC) serves as an ideal system to study the shape of the local ECP involving several competing scattering mechanisms under discussion [4] , [5] , [18] . The atomic scale structure encountered at such a ML–BL junction is depicted in Fig. 1b . A graphene sheet from the ML side starts to coat an underlying additional graphene sheet on the BL side. This configuration is known to be caused by the thermal decomposition of SiC during growth of graphene, which always leads to new graphene layers under preceding sheets [19] , [20] . For the ML–BL junction, a change in electronic properties occurs directly at the structural boundary (blue vertical line in Fig. 1b ). It has been proposed that the wave function mismatch at the junction leads to a reduced transmission probability of ML states into the BL region [4] , [5] , [7] . A highly localized jump of the ECP in ref. 5 is explicitly attributed to this dominant scattering mechanism at a ML–BL boundary. Moreover, at the junction, the continuous upper sheet is bent and detached from the substrate (light blue area in Fig. 1b ). A similar configuration is encountered when a ML graphene sheet covers a substrate step (ML–ML junction). In this case, the detachment of the graphene sheet and its consequently changed local electron density was theoretically found to be the dominating contribution to the resistance [18] . 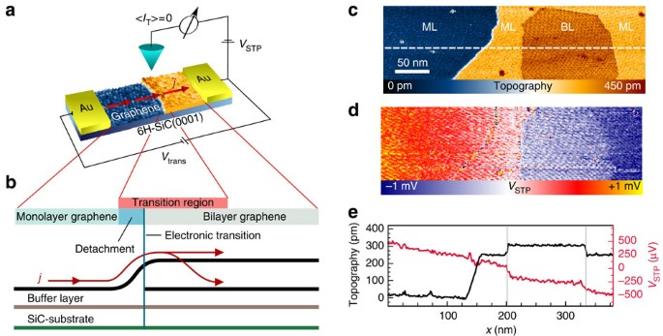Figure 1: Scanning tunnelling potentiometry and the graphene monolayer–bilayer junction. (a) Schematic of the setup of our scanning tunnelling potentiometry experiment. The epitaxially grown graphene sample is contacted with gold in two-point geometry. The voltagenecessary to compensate a net tunnel currentITis recorded and mapped. It represents the voltage drop along the sample induced by the voltageVTrans.jis the current density in the sample. (b) Sketch of the structural transition from monolayer (ML) into bilayer (BL) graphene and the consequences for electron transport. The upper graphene layer is continuous and connects to the lower bilayer sheet via interlayer coupling. The electrical resistance of the junction is caused by the detachment of the graphene sheet from the underlying substrate and the transition of the electronic states from monolayer- to bilayer-like. Although the former leads to a voltage drop directly at the step, our experiments show that the transition of the electrons into the bilayer happens on a nanometre scale. (c) Large scale topography and (d) the respective potential map forVSTP. (e) Section along the white line incthat reveals the delocalized linear voltage drop on the monolayer and bilayer sheets, whereas a distinct localized voltage drop is found at the ML/BL-interfaces (marked with grey lines) and a less prominent one at the substrate step covered with a ML graphene sheet. (imaging conditions:IT=0.2 nA,VBias=−30 mV,j=12 Am−1). Figure 1: Scanning tunnelling potentiometry and the graphene monolayer–bilayer junction. ( a ) Schematic of the setup of our scanning tunnelling potentiometry experiment. The epitaxially grown graphene sample is contacted with gold in two-point geometry. The voltage necessary to compensate a net tunnel current I T is recorded and mapped. It represents the voltage drop along the sample induced by the voltage V Trans . j is the current density in the sample. ( b ) Sketch of the structural transition from monolayer (ML) into bilayer (BL) graphene and the consequences for electron transport. The upper graphene layer is continuous and connects to the lower bilayer sheet via interlayer coupling. The electrical resistance of the junction is caused by the detachment of the graphene sheet from the underlying substrate and the transition of the electronic states from monolayer- to bilayer-like. Although the former leads to a voltage drop directly at the step, our experiments show that the transition of the electrons into the bilayer happens on a nanometre scale. ( c ) Large scale topography and ( d ) the respective potential map for V STP . ( e ) Section along the white line in c that reveals the delocalized linear voltage drop on the monolayer and bilayer sheets, whereas a distinct localized voltage drop is found at the ML/BL-interfaces (marked with grey lines) and a less prominent one at the substrate step covered with a ML graphene sheet. (imaging conditions: I T =0.2 nA, V Bias =−30 mV, j =12 Am −1 ). Full size image Large scale STP In Fig. 1c , the topography of a typical structure of our epitaxial graphene samples is shown. The simultaneously acquired potential map in Fig. 1d shows the voltage drop on a scale of several 100 nm caused by a current density in the graphene layer of j =12 Am −1 . (For evaluation of low-temperature STP data, see Supplementary Note 1 and Supplementary Fig. 1 ). It reflects the scattering mechanisms discussed above. A section along the white dashed line of Fig. 1c of both topography and potential map shown in Fig. 1e reveals the large voltage drop associated with the ML/BL interface. In the following, we will resolve the transition of the ECP on the atomic scale. Extent and shift of the electrochemical potential In Fig. 2 , a topography map ( Fig. 2a , Supplementary Fig. 2 ) and the corresponding potential map ( Fig. 2b ) that focus on a ML/BL step with higher resolution is shown. In the potential map, we find a distinct lateral extension of the ML potential into the BL with respect to the localized topographic step (black line). The onset of this voltage drop is located at the topographic step while its final value is found several nanometres inside the bilayer. This becomes even more evident in Fig. 2c , where we show sections along the coloured lines indicated in Fig. 2a . The difference between the midpoint of the step in the topography and the end of the potential is indicated for the pink line by the blue-shaded area, which is found to be ~3 nm wide. This difference holds also for the other sections or becomes even larger (purple section). Up to its maximum, the potential rises continuously. The smooth potential slope and its spatial extent are not expected from previous models for the ML/BL interface that predict the potential drop directly at the electronic transition [5] . To prove that this electronic transition between ML and BL is located at the topographic step, we have carried out a spectroscopy measurement shown in Fig. 2d . In the range of ±100 mV, it shows the differential conductance for n-doped SiC-graphene for both ML and BL graphene consistent with others [18] . Within the experimental resolution of 0.4 nm, topography and spectroscopy are both in perfect synchronicity at the Fermi-energy ( Fig. 2e ). This shows that in contrast to the large extension of the voltage drop at the ML/BL interface, the measured electronic spectra change abruptly at the step. Moreover, tip jumping artefacts can be excluded ( Supplementary Note 2 , Supplementary Fig. 3 ). 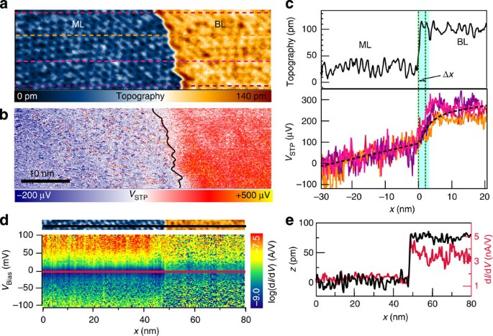Figure 2: High-resolution potentiometry at a ML/BL junction. (a) Topography (imaging conditions:IT=0.2 nA,VBias=−50 mV,j=10 Am−1) and (b) corresponding potential map forVSTP. The black line indicates the position of the step ina. (c) Data sections comparing the topography and voltage drop along the lines ina. All sections (average of 10 lines) have been shifted laterally, so that the corresponding step is located atx=0 nm for all sections. The green dotted lines indicate the lateral offset Δxbetween the FWHM value points of the topography and the potential for the pink curve. The blue-shaded area indicates the distance to the maximum of the voltage drop. The drop is shifted into the bilayer region with a smooth evolution of the potential, which is varying on a local scale (see purple and yellow section). The black dotted line shows the fit of the voltage drop to the classical model as described in the text. (d) Scanning tunnelling spectroscopy (STS) measurement crossing the ML/BL junction inaas indicated at the top. (e) Section along the black and red lines indcomparing the topography with the spectroscopy at 0 mV. The transition in the STS is strictly located at the topographic position of the step (imaging conditions:IT=0.35 nA,VBias=−100 mV). Figure 2: High-resolution potentiometry at a ML/BL junction. ( a ) Topography (imaging conditions: I T =0.2 nA, V Bias =−50 mV, j =10 Am −1 ) and ( b ) corresponding potential map for V STP . The black line indicates the position of the step in a . ( c ) Data sections comparing the topography and voltage drop along the lines in a . All sections (average of 10 lines) have been shifted laterally, so that the corresponding step is located at x =0 nm for all sections. The green dotted lines indicate the lateral offset Δ x between the FWHM value points of the topography and the potential for the pink curve. The blue-shaded area indicates the distance to the maximum of the voltage drop. The drop is shifted into the bilayer region with a smooth evolution of the potential, which is varying on a local scale (see purple and yellow section). The black dotted line shows the fit of the voltage drop to the classical model as described in the text. ( d ) Scanning tunnelling spectroscopy (STS) measurement crossing the ML/BL junction in a as indicated at the top. ( e ) Section along the black and red lines in d comparing the topography with the spectroscopy at 0 mV. The transition in the STS is strictly located at the topographic position of the step (imaging conditions: I T =0.35 nA, V Bias =−100 mV). Full size image In total, we evaluated the voltage drop at 13 independent ML–BL boundaries in a quantitative manner including configurations with and without an underlying substrate step. As a quantitative measure ( Supplementary Note 3 , Supplementary Table 1 ), we use the lateral mean offset ‹Δ x › between the full width at half maximum value points of the topographic and the full width at half maximum value points of the potential transition (green lines in Fig. 2c ). The result of this evaluation is shown in Fig. 3 . On average, we obtain ‹Δ x › ML/BL =+2.0±0.5 nm. The full spatial extension of the potential drop is ‹ L › Δ V =4.0±1.3 nm and the voltage drop is therefore almost completely located in the bilayer region. To check that this shift is particularly connected to the ML/BL interface, we analysed substrate steps covered by a single continuous layer of graphene (ML/ML junction). In agreement with other works [4] , [7] , we find that the detachment of the sheet at a substrate step causes a voltage drop, but we do not observe a lateral shift leading to ‹Δ x › ML/ML =0.3±0.4 nm. This shows that the extended potential shift is connected to the electronic transition between ML and BL and not to the presence of the step itself. 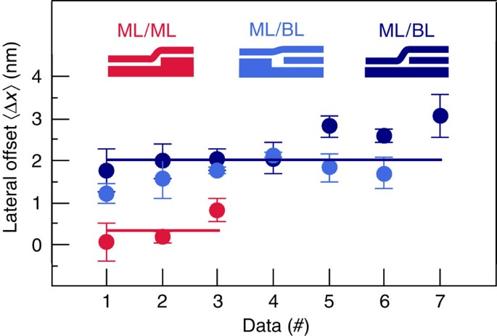Figure 3: Statistic of the lateral offset. Statistic of the lateral offset ‹Δx› between the transition in the topography and the transport map. Error bars show the standard deviation. It reveals an offset into the bilayer for different types of ML/BL-steps in contrast to ML/ML-substrate steps (red). For the ML/BL-steps, two different configurations have been observed, one involving an additional SiC-substrate step (light blue) and one without an additional step (dark blue). Figure 3: Statistic of the lateral offset. Statistic of the lateral offset ‹Δ x › between the transition in the topography and the transport map. Error bars show the standard deviation. It reveals an offset into the bilayer for different types of ML/BL-steps in contrast to ML/ML-substrate steps (red). For the ML/BL-steps, two different configurations have been observed, one involving an additional SiC-substrate step (light blue) and one without an additional step (dark blue). Full size image Separation of different scattering contribution Besides the electronic transition, each ML/BL junction contains also a detachment from the substrate. The additional scattering contribution should be distinguishable from the interlayer coupling at least for certain configurations of the junction. This becomes visible for the ML/BL boundary shown in Fig. 4 . Here, the lateral section of the ECP depicted in Fig. 4c clearly reveals a two-step potential drop. First, a small drop Δ V 1 is seen directly at the position of the step and second, a large drop Δ V 2 occurs deep within the bilayer. We attribute Δ V 1 to the detachment as observed for ML/ML-surface steps and Δ V 2 to the ML/BL-interlayer coupling ( Fig. 4d ) as discussed for the step in Fig. 2 . 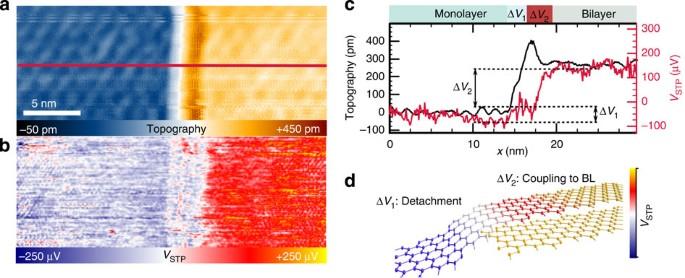Figure 4: Resolving different scattering components. (a) Topography of a ML/BL boundary and (b) the corresponding change in the ECPVSTP(imaging conditions:IT=0.24 nA,VBias=−40 mV,j=4 Am−1). (c) Sections along the line ina. Two distinct voltage drops, ΔV1directly at the step and ΔV2again in the bilayer are visible. (d) Scattering processes for the potential drops inc. ΔV1is caused by the detachment of the sheet from the substrate reducing the doping. The major contribution ΔV2is again shifted into the bilayer and results from the interlayer coupling. Figure 4: Resolving different scattering components. ( a ) Topography of a ML/BL boundary and ( b ) the corresponding change in the ECP V STP (imaging conditions: I T =0.24 nA, V Bias =−40 mV, j =4 Am −1 ). ( c ) Sections along the line in a . Two distinct voltage drops, Δ V 1 directly at the step and Δ V 2 again in the bilayer are visible. ( d ) Scattering processes for the potential drops in c . Δ V 1 is caused by the detachment of the sheet from the substrate reducing the doping. The major contribution Δ V 2 is again shifted into the bilayer and results from the interlayer coupling. Full size image To explain the shift of the voltage drop at ML/BL junctions into the bilayer side, we recall its geometry as shown in Fig. 1b . The monolayer sheet is continuously connected to the upper bilayer sheet. As known from multilayer graphene and graphite, this upper bilayer sheet is connected to the lower bilayer sheet via a significantly higher interlayer resistivity compared with the in-plane resistivity [21] , [22] . In addition to the higher c -axis resistivity, the electron density is reduced in the upper layer due to distance-dependent buffer-layer doping [23] , [24] and therefore its in-plane resistance also is increased [17] . Theoretically, this layer-dependent conductivity has been demonstrated in a gated bilayer; as for distinct voltages perpendicular to the sheet, the current in one layer can even be tuned to zero [25] . Accordingly, the difference in electron density of the second layer in combination with the high interlayer resistivity leads to a bottleneck for electron transport. The interlayer hopping process necessary to populate the lower sheet with higher electron density extends the effective transport barrier spatially into the bilayer. To model this situation, we use a resistor network, which has already been successfully applied to local transport experiments [2] , [4] , [26] , as well as an analytical model derived for voltage drops at interfaces in scanning probe experiments [27] ( Supplementary Note 4 , Supplementary Figs 4–6 ). Both models consider the problem of electron transfer with a contact resistance, which treats the bottom sheet of the bilayer as a contact to the top one. The best fit with this model is shown by the black dotted line in Fig. 2c . Though we only apply a classical model neglecting quantum coherence, the results reproduce the observed shape and length scale of the ECP. Moreover, the model allows to extract a contact resistance of R C =4.2 × 10 −10 Ω cm 2 which is reasonable when compared with c -axis resistivity in graphene and graphite ( Supplementary Note 4 ). A comprehensive explanation for the extension of the ECP into the BL side should include the decaying states present on the bilayer according to Nakanishi et al . [28] This weak coupling determines the local ECP in the same way as was proposed by theory for single molecules. Here, a reduction in orbital overlap leads to an effective potential barrier for electron transport inside a molecule and at its contacts [9] , [10] . The shift of the potential drop into the bilayer indicates a better coupling of the junction region to the monolayer than to the bilayer side. This picture of electron transport also becomes important when graphene is considered as an electrode material in molecular junctions [29] . The results obtained from Fig. 4 not only show that the transition region contains more than one scattering mechanism, but also that their relative magnitude can be resolved by STP on the scale of few nanometres. Moreover, in the region between the two potential drops, the potential does not change significantly ( Fig. 4c ). After the first increase in potential Δ V 1 due to the detachment of the graphene, it takes a certain distance before the onset of Δ V 2 . Since in the topography the wrinkle structure is located in this region, we hypothesize that the bending of the upper sheet as well as other mechanisms located in this region (for example, interface states) are less relevant than the electronic ML/BL transition. This would fit to theoretical results showing that bending has a negligible effect on the resistance of graphene [18] . Up to now highly spatially resolved information of a transition region of the electrochemical potential in the presence of a localized barrier was accessible only by theoretical treatments [1] , [9] , [10] , [12] , [13] , [14] , [15] , [16] . Dissecting experimentally, the spatial evolution of the ECP with Angstrom resolution at low temperature opens a new way to non-thermal equilibrium, molecular and coherent quantum transport phenomena. This includes conceptually open questions like the transition from a quantum mechanical description to diffusive scattering. Sample preparation Samples with epitaxial mono- and bilayer graphene are prepared by thermal decomposition of n-doped 6H-SiC(0001) [30] at T =1400–1600 °C under ultra-high vacuum (UHV, 10 −10 mbar).The samples (2 mm × 7 mm) are electrically contacted ex situ with gold contacts of 100 nm thickness by thermal evaporation through a shadow mask. After reinsertion into the UHV chamber, the samples are heated up to 350 °C for 30 min to eliminate surface contaminations before they are transferred in situ to a homebuilt low-temperature scanning tunnelling microscope. All the measurements were performed at 6 K sample temperature. Scanning probe measurements STP measurements are taken at every image point by adjusting the ECP at the tip at fixed tip-sample distance. For STP, the applied bias voltage is switched off while only the transport potential across the sample remains. The potential at the tip is adjusted in a way that the tunnelling current I T =0. Subsequently, the voltage necessary to compensate the net tunnel current is recorded (See Fig. 1a ). This voltage has been referred to as the local ECP, which is here inherently defined by the STP method [2] , [6] , [31] . The measurements are made at different values of the electron current in the sample plane, especially at zero and forward and reversed current as defined by the potential applied to the sample contacts. The details of our specific setup are published elsewhere [31] . How to cite this article: Willke, P. et al . Spatial extent of a Landauer residual-resistivity dipole in graphene quantified by scanning tunnelling potentiometry. Nat. Commun. 6:6399 doi: 10.1038/ncomms7399 (2015).